Optogenetic astrocyte activation modulates response selectivity of visual cortex neuronsin vivo Astrocytes play important roles in synaptic transmission and plasticity. Despite in vitro evidence, their causal contribution to cortical network activity and sensory information processing in vivo remains unresolved. Here we report that selective photostimulation of astrocytes with channelrhodopsin-2 in primary visual cortex enhances both excitatory and inhibitory synaptic transmission, through the activation of type 1a metabotropic glutamate receptors. Photostimulation of astrocytes in vivo increases the spontaneous firing of parvalbumin-positive (PV + ) inhibitory neurons, while excitatory and somatostatin-positive (SOM + ) neurons show either an increase or decrease in their activity. Moreover, PV + neurons show increased baseline visual responses and reduced orientation selectivity to visual stimuli, whereas excitatory and SOM + neurons show either increased or decreased baseline visual responses together with complementary changes in orientation selectivity. Therefore, astrocyte activation, through the dual control of excitatory and inhibitory drive, influences neuronal integrative features critical for sensory information processing. Astrocytes are emerging as the central elements of brain circuits involved in different aspects of neuronal physiology relevant for brain functions [1] , [2] . Accumulating evidence has shown that astrocytes play important roles in synaptic function by releasing glutamate and other gliotransmitters [3] , [4] , [5] , [6] , [7] . Despite these in situ studies, the role of astrocytes in cortical functions in vivo is poorly understood. Although cortical astrocytes are known to respond to neural activity in vivo [8] , [9] , [10] , [11] , [12] , it has proven difficult to separate their activation from that of nearby neurons, and thus elementary questions about their impact on neuronal networks and the coding and representation of information are still unresolved. The primary visual cortex is the neocortical area that receives visual input from the retina. It is well known that visual cortex neurons show complex visual property features, such as orientation preference or ocular dominance [13] . Recently, astrocytes have been shown to respond to visual stimuli, and their responses can be tuned based on visual stimulus features including orientation and spatial frequency [9] . Although astrocytes respond to visual sensory stimuli [8] , [9] , their role in the processing of sensory information is poorly known. Here we show that selective photostimulation of astrocytes with channelrhodopsin-2 (ChR2) in V1 increases both excitatory and inhibitory synaptic transmissions, through the activation of type 1a metabotropic glutamate receptors. Furthermore, optical activation of astrocytes in vivo impact the spontaneous firing rate of cortical neurons—that is, enhances parvalbumin-positive (PV + ) inhibitory neurons—while excitatory and somatostatin-positive (SOM + ) neurons show either an increase or decrease in their activity. In addition, PV + neurons show increased baseline visual responses and reduced orientation selectivity to visual stimuli, whereas excitatory and SOM + neurons show either increased or decreased baseline visual responses together with complementary changes in orientation selectivity. Therefore, optical activation of astrocytes influences neuronal response features in primary visual cortex (V1) critical for sensory information processing. Optical astrocyte activation increases synaptic activity in V1 We first assessed the response levels of astrocytes in V1 in vivo to sensory drive by recording their visually driven intracellular Ca 2+ responses when stimulated with drifting gratings [8] , [9] ( Supplementary Fig. 1 ; increase in fluorescence area post-visual stimulation measured as the Ca 2+ area index 0.56±0.14 (mean±s.e.m. for all data shown; P <0.001, Wilcoxon test; n =22 astrocytes from two mice; see Methods Equation (1)). Then, in order to causally understand the contribution of astrocyte activation to cortical networks, astrocytes were selectively manipulated using ChR2 (refs 14 , 15 ). The specificity of ChR2 expression in astrocytes induced by viral vectors was confirmed ( Fig. 1a ; ChR2 driven by a glial fibrillary acidic protein (GFAP) promoter, Supplementary Figs 2 and 3 ; see Methods), and light stimulation used to robustly induce astrocyte Ca 2+ elevation in cultured cells ( Supplementary Fig. 2 ) and V1 cortical slices (Ca 2+ area index 0.43±0.06; P <0.001, Wilcoxon test; n =59 astrocytes; Fig. 1c ; Supplementary Fig. 3 ). The functional consequences of selective astrocyte activation on neuronal activity were analysed by recording synaptic activity in layer 2/3 pyramidal neurons of V1. Astrocyte photostimulation transiently increased the frequency of spontaneous excitatory postsynaptic currents (EPSCs; seven out of nine cells; 1.76±0.52 Hz pre- versus 2.63±0.62 Hz post-astrocyte stimulation, P =0.0017, t- test; mean increase 194.6±30.31% of control; P =0.014, t -test; n =9 neurons; Fig. 1e–g ), without affecting their amplitude (7.24±0.91 pA pre- versus 7.06±1.02 pA post-astrocyte stimulation, P =0.69, t- test; the mean increase 98.47±6.99% of control, P =0.92, t -test; Fig. 1f,g ). The analysis of astrocyte Ca 2+ signals showed that they preceded the changes observed in EPSCs induced by ChR2 stimulation ( Supplementary Fig. 3h ). Similar to EPSCs, the spontaneous inhibitory synaptic currents (IPSCs) increased after ChR2-astrocyte stimulation, showing an enhancement of their frequency (seven out of 10 cells; 1.26±0.20 Hz pre- versus 2.03±0.27 Hz post-astrocyte stimulation, P =0.004, t- test; the mean increase 180.98±19.48% of control, P =0.002, t- test; n =10 neurons; Fig. 1h–j ), without changes in the amplitude of synaptic currents (20.25±2.37 pA pre- versus 20.68±3.46 pA post-astrocyte stimulation, P =0.83, t- test; the mean increase 98.28±10.69% of control, P =0.92, t -test; Fig. 1i,j ). Therefore, photostimulation of astrocytes modulates synaptic transmission in cortical neurons by increasing the frequency of both excitatory and IPSCs. No changes in astrocyte Ca 2+ signalling and EPSCs were observed in contralateral non-infected slices after light stimulation ( Supplementary Fig. 4 ), indicating that these phenomena were induced by selective optogenetic activation of astrocytes rather than by nonspecific action of light. In addition, neuronal membrane potentials did not show shifts that were synchronized with astrocyte photostimulation, indicating that a direct action of photostimulation on neurons was absent (0.34±0.87 mV change during photostimulation; n =6; P =0.27, t- test; Fig. 1d ). 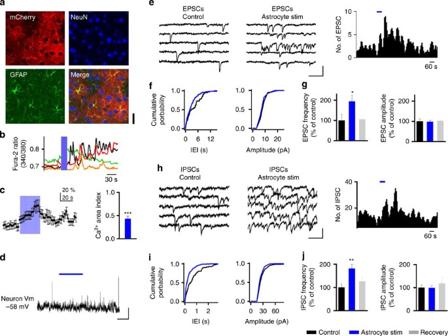Figure 1: Selective stimulation of ChR2-transfected astrocytes induces enhancement of synaptic transmission in layer 2/3 of V1. (a) Immunocytochemical localization of ChR2–mCherry, NeuN and GFAP in V1 cortical slices. Note the selective expression of ChR2–mCherry in astrocytes (bottom). Scale bar, 15 μm. (b) Astrocyte Ca2+signals evoked by ChR2 stimulation (20 Hz, 20 s; blue bar). (c) Population astrocyte Ca2+signal versus time evoked by ChR2 stimulation (20 Hz, 30 s; blue bar) and Ca2+area index (n=59 astrocytes from 7 slices from three mice). ***P<0.001; Wilcoxon Test. (d) Representative neuron membrane potential recording during astrocyte photostimulation (20 Hz, 60 s; blue horizontal bar). Scale bar, 4 mV, 30 s. (e,h) Representative recordings from 2/3 layer neurons of spontaneous excitatory currents (EPSCs,e) and IPSCs (h) before (Control) and after astrocyte stimulation. Scale bar, 10 pA, 200 ms for EPSCs; 40 pA, 200 ms for IPSCs. Right, histogram of number of EPSCs and IPSCs versus time (bin width 10 s) before and after astrocyte stimulation (20 Hz, 60 s; blue horizontal bar). (f,i) Cumulative probability plots for inter-event interval (bin width 20 ms) and synaptic current amplitude (bin width 3pA) before and after astrocyte stimulation (black and blue traces, respectively) from neurons shown ine,h. (g,j) Relative changes in EPSC and IPSC frequency and amplitude in control, during astrocyte stimulation and 10-min post stimulation (recovery) (EPSCs,n=9 neurons; IPSCs,n=10 neurons). *P<0.05, **P<0.01; Two-tailed Student’st-test. Error bars indicate s.e.m. Figure 1: Selective stimulation of ChR2-transfected astrocytes induces enhancement of synaptic transmission in layer 2/3 of V1. ( a ) Immunocytochemical localization of ChR2–mCherry, NeuN and GFAP in V1 cortical slices. Note the selective expression of ChR2–mCherry in astrocytes (bottom). Scale bar, 15 μm. ( b ) Astrocyte Ca 2+ signals evoked by ChR2 stimulation (20 Hz, 20 s; blue bar). ( c ) Population astrocyte Ca 2+ signal versus time evoked by ChR2 stimulation (20 Hz, 30 s; blue bar) and Ca 2+ area index ( n =59 astrocytes from 7 slices from three mice). *** P <0.001; Wilcoxon Test. ( d ) Representative neuron membrane potential recording during astrocyte photostimulation (20 Hz, 60 s; blue horizontal bar). Scale bar, 4 mV, 30 s. ( e , h ) Representative recordings from 2/3 layer neurons of spontaneous excitatory currents (EPSCs, e ) and IPSCs ( h ) before (Control) and after astrocyte stimulation. Scale bar, 10 pA, 200 ms for EPSCs; 40 pA, 200 ms for IPSCs. Right, histogram of number of EPSCs and IPSCs versus time (bin width 10 s) before and after astrocyte stimulation (20 Hz, 60 s; blue horizontal bar). ( f,i ) Cumulative probability plots for inter-event interval (bin width 20 ms) and synaptic current amplitude (bin width 3pA) before and after astrocyte stimulation (black and blue traces, respectively) from neurons shown in e , h . ( g , j ) Relative changes in EPSC and IPSC frequency and amplitude in control, during astrocyte stimulation and 10-min post stimulation (recovery) (EPSCs, n =9 neurons; IPSCs, n =10 neurons). * P <0.05, ** P <0.01; Two-tailed Student’s t- test. Error bars indicate s.e.m. Full size image As astrocytes can evoke changes in the presynaptic release of neurotransmitters [3] , [6] , [12] , [16] , [17] , we examined the effects of astrocyte activity on miniature EPSCs (mEPSCs; isolated in the presence of Tetrodotoxin (TTX), 1 μM). mEPSCs showed an increase in frequency after astrocyte stimulation (11 out of 15 cells; 0.73±0.17 pre- versus 1.07±0.26 post-astrocyte stimulation; mean increase 150.75±8.13% of control; P <0.001, t- test; n =15; Fig. 2a,c ), without significant changes in amplitude (7.44±0.62 pA pre- versus 7.52±0.80 pA post-astrocyte stimulation; mean increase 98.80±2.80% of control; P =0.67, t- test; Fig. 2c ). In addition, astrocyte stimulation affected miniature IPSCs (mIPSCs), increasing mIPSC frequency (six out of eight cells; 165.07±17.77% of control; P =0.008, t- test; n =8) with no change in their amplitude (112.60±8.26% of control; P =0.57, t- test; n =8; Fig. 2c ). Thus, these data indicate that photostimulation of astrocytes induces a short-term enhancement of both spontaneous and miniature excitatory and inhibitory synaptic transmissions, increasing neurotransmitter release principally through presynaptic mechanisms. 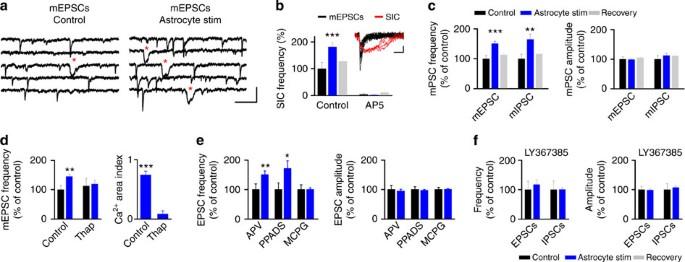Figure 2: Astrocyte-induced enhancement of synaptic transmission is mediated by mGluR activation. (a) Whole-cell recordings from 2/3 layer neurons of mEPSCs and SICs (red asterisks), showing an increase in frequency of mEPSC and SICs after astrocyte optogenetic stimulation. Scale bar, 15pA, 200 ms. (b) Relative changes of SIC frequency before (control; black), during astrocyte stimulation (blue) and after stimulation (recovery; grey) before and after perfusion of AP5 (50 μM;n=5).Inset right, representative traces of mEPSCs (black traces) and SICs (red traces) from neuron shown ina. Scale bar, 5pA, 20 ms. (c) Relative changes of mEPSC (n=15) and mIPSC (n=8) frequency and amplitude before (Control), during astrocyte stimulation, and 10-min post stimulation (recovery). (d) Relative changes of mEPSC frequency before (control) and after astrocyte stimulation in the presence of thapsigargin (1 μM;n=6). **P<0.01; two-tailed Studentt-test. Ca2+area index following ChR2 stimulation before and after thapsigargin (n=32 astrocytes from four slices from two mice). ***P<0.001; Wilcoxon test. (e) Relative changes of spontaneous EPSC frequency and amplitude before (control) and after astrocyte stimulation in the presence of AP5 (50 μM;n=10), PPADS (30 μM;n=7) and MCPG (0.8 mM;n=13), respectively. (f) Relative changes of spontaneous EPSC (n=9) and IPSC (n=7) frequency and amplitude evoked by astrocyte stimulation in the presence of LY367385 (100 μM). *P<0.05, **P<0.01, ***P<0.001; two-tailed Student’st-test. Error bars indicate s.e.m. Figure 2: Astrocyte-induced enhancement of synaptic transmission is mediated by mGluR activation. ( a ) Whole-cell recordings from 2/3 layer neurons of mEPSCs and SICs (red asterisks), showing an increase in frequency of mEPSC and SICs after astrocyte optogenetic stimulation. Scale bar, 15pA, 200 ms. ( b ) Relative changes of SIC frequency before (control; black), during astrocyte stimulation (blue) and after stimulation (recovery; grey) before and after perfusion of AP5 (50 μM; n =5). Inset right , representative traces of mEPSCs (black traces) and SICs (red traces) from neuron shown in a . Scale bar, 5pA, 20 ms. ( c ) Relative changes of mEPSC ( n =15) and mIPSC ( n =8) frequency and amplitude before (Control), during astrocyte stimulation, and 10-min post stimulation (recovery). ( d ) Relative changes of mEPSC frequency before (control) and after astrocyte stimulation in the presence of thapsigargin (1 μM; n =6). ** P <0.01; two-tailed Student t -test. Ca 2+ area index following ChR2 stimulation before and after thapsigargin ( n =32 astrocytes from four slices from two mice). *** P <0.001; Wilcoxon test. ( e ) Relative changes of spontaneous EPSC frequency and amplitude before (control) and after astrocyte stimulation in the presence of AP5 (50 μM; n =10), PPADS (30 μM; n =7) and MCPG (0.8 mM; n =13), respectively. ( f ) Relative changes of spontaneous EPSC ( n =9) and IPSC ( n =7) frequency and amplitude evoked by astrocyte stimulation in the presence of LY367385 (100 μM). * P <0.05, ** P <0.01, *** P <0.001; two-tailed Student’s t -test. Error bars indicate s.e.m. Full size image The ability of ChR2 to stimulate astrocyte gliotransmission was also confirmed by recording glutamatergic N-methyl-D-aspartate (NMDA) receptor-mediated inward currents (‘slow inward currents’ or SICs; see Methods) [8] , [18] , [19] , [20] . Indeed, astrocyte photostimulation induced an increase in the frequency of these currents (3.20±1.10 min −1 pre- versus 5.02±1.36 min −1 post-astrocyte stimulation, P =0.0013, t- test; mean increase 181.19±16.79% of control; P <0.001, t- test; n =10; Fig. 2a,b ), which was abolished in the presence of the NMDA antagonist AP5 (50 μM; n =5; Fig. 2b ). Astrocyte Ca 2+ and metabotropic glutamate receptor 1a boost neuronal activity To further assess the relationship between astrocyte Ca 2+ signals and the enhancement of synaptic activity, we perfused thapsigargin (1 μM; an inhibitor of the sarco/endoplasmic reticulum Ca 2+ ATPase). Thapsigargin blocked both the increase in astrocyte Ca 2+ signal in cultured astrocytes and cortical slices ( Fig. 2d and Supplementary Fig. 2d ; cf . [14] ). In addition, mEPSC frequency induced by ChR2 stimulation ( Fig. 2d ) was abolished by thapsigargin, without affecting basal levels of synaptic transmission ( Supplementary Fig. 3f ), supporting the proposal that astrocytic Ca 2+ elevation induces changes in synaptic transmission. Besides other active substances, astrocytes release glutamate and ATP [21] that can be also evoked by optical stimulation [14] , [22] , [23] ; thus, we evaluated the role of these gliotransmitters in the enhancement of synaptic transmission. The increase in spontaneous EPSCs induced by astrocyte stimulation was unaffected in the presence of NMDA antagonist AP5 (50 μM; mean increase 150.98±12.90% of control; P =0.003, t- test; n =10; Fig. 2e ), as well as in the presence of purinergic P2Y receptor antagonist PPADS (100 μM; mean increase 172.18±25.87% of control; P =0.038, t- test; n =7; Fig. 2e ), indicating that the enhancement of EPSCs was independent of NMDA receptor activation or P2Y purinergic signalling. In the hippocampus and cerebellum, astrocytes influence synaptic transmission through activation of group I mGluRs [6] , [12] , [16] , [22] . Thus, we first analysed the contribution of mGluRs to these responses. MCPG (0.8 mM; a group I and II mGluR antagonist) inhibited the facilitation of EPSC frequency (mean increase 100.04±6.19% of control; P =0.99, t- test; n =13; Fig. 2e ). Selective activation of mGluR1a, a subtype of group I mGluRs, has been related to facilitation of both excitatory and inhibitory synaptic transmissions in different cortical areas [24] , [25] , [26] . Blockage of mGluR1a with the antagonist LY367385 (100 μM) abolished the increase in both EPSC (mean increase 117.24±16.0% of control; P =0.31, t -test; n =9) and IPSC frequency (mean increase 100.25±6.63% of control; P =0.97, t -test; n =7; Fig. 2f ) induced by astrocyte photostimulation, indicating that astrocytes enhance excitatory and inhibitory synaptic transmissions in V1 cortical neurons through presynaptic mGluR1a activation. In addition, mEPSCs were also recorded in identified cortical inhibitory neuron subtypes, including PV + and SOM + neurons ( Fig. 3 ). In these cells, astrocyte stimulation evoked an increase in mEPSC frequency mediated by mGluR1a activation ( Fig. 3c,d ), showing that astrocyte activity directly enhanced excitatory transmission in cortical networks affecting both pyramidal and inhibitory cells. 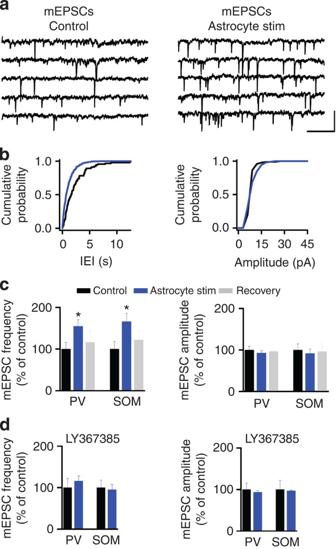Figure 3: Selective stimulation of ChR2-transfected astrocytes induces enhancement of miniature excitatory synaptic transmission in PV+and SOM+neurons. (a) Representative recordings from PV+neurons of mEPSCs before (Control) and after astrocyte stimulation. Scale bar, 15 pA, 200 ms. (b) Cumulative probability plots for inter-event interval (bin width 20 ms) and synaptic current amplitude (bin width 3 pA) before and after astrocyte stimulation (black and blue traces, respectively) from neuron shown ina. (c) Relative changes in mEPSC frequency and amplitude in control, during astrocyte stimulation and 10-min post stimulation (recovery) for PV+neurons (n=9) and SOM+neurons (n=5). (d) Relative changes of mEPSC frequency and amplitude evoked by astrocyte stimulation in the presence of LY367385 (100 μM; PV+neurons,n=7; SOM+neurons,n=5). *P<0.05; two-tailed Student’st-test. Error bars indicate s.e.m. Figure 3: Selective stimulation of ChR2-transfected astrocytes induces enhancement of miniature excitatory synaptic transmission in PV + and SOM + neurons. ( a ) Representative recordings from PV + neurons of mEPSCs before (Control) and after astrocyte stimulation. Scale bar, 15 pA, 200 ms. ( b ) Cumulative probability plots for inter-event interval (bin width 20 ms) and synaptic current amplitude (bin width 3 pA) before and after astrocyte stimulation (black and blue traces, respectively) from neuron shown in a . ( c ) Relative changes in mEPSC frequency and amplitude in control, during astrocyte stimulation and 10-min post stimulation (recovery) for PV + neurons ( n =9) and SOM + neurons ( n =5). ( d ) Relative changes of mEPSC frequency and amplitude evoked by astrocyte stimulation in the presence of LY367385 (100 μM; PV + neurons, n =7; SOM + neurons, n =5). * P <0.05; two-tailed Student’s t -test. Error bars indicate s.e.m. Full size image Astrocytes increase spontaneous neuronal activity in vivo We next investigated the role of astrocytes in regulating the activity and dynamics of V1 neurons and networks in vivo . Astrocyte Ca 2+ signals and neuronal activity were monitored in layer 2/3 of V1 ( Fig. 4 ) in anaesthetised mice transduced with GFAP-ChR2. Two-photon calcium imaging of ChR2-expressing astrocytes in vivo showed robust intracellular Ca 2+ elevations (Ca 2+ area index 0.66±0.03; P <0.001, Wilcoxon test; n =33 astrocytes from three mice; Fig. 4b,c ). To investigate the consequences of astrocyte photostimulation on excitatory and inhibitory transmissions in vivo , we used transgenic mice to carry out visualized cell-attached electrophysiological recordings from targeted neuron types, including excitatory neurons (in thy1-GFP-S mice) and PV + inhibitory neurons (in PV-tdTomato mice; Fig. 4d,e ). First, we monitored the spontaneous firing rate before and after astrocyte stimulation. Excitatory neurons showed an overall increase in their firing rate after astrocyte stimulation ( Fig. 4f,j ), although with a wide range of effects ( Fig. 4h ). Spontaneous firing activity was significantly reduced in a subset of excitatory cells (13 of 45 neurons; 29%), while it was increased in other cells ( n =18 of 45 neurons; 36%; Fig. 4h ). Interestingly, PV + neurons also showed a significant increase in their spontaneous firing rate ( n =11 of 18 neurons; 61%; Fig. 4g,j ); however, none of the cells showed a decrease in their activity after astrocyte stimulation ( Fig. 4i ). These results support and extend the slice data, demonstrating that activation of astrocytes in vivo regulates neuronal activity by increasing excitatory drive to PV + neurons, and either by increasing or decreasing net drive to excitatory neurons. 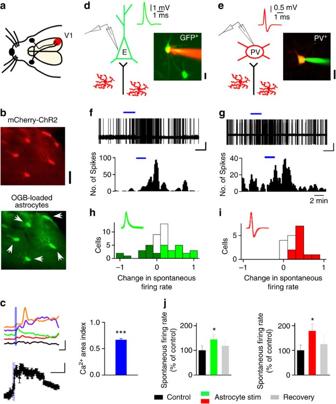Figure 4: Astrocytes modulate spontaneous activity of PV+and excitatory visual cortex neuronsin vivo. (a) Schematic illustration of the visual pathway in mice, andin vivoChR2–mCherry expression in V1 for calcium imaging and electrophysiological recordings. (b) Representative fluorescence images of ChR2–mCherry-expressing astrocytes bulk-loaded with OGB (arrows). Scale bar, 40 μm. (c)Up, representative astrocyte Ca2+signals evoked by ChR2 stimulation (5 Hz, 20 s; blue bar). Scale bar, 40%, 60 s.Down, population astrocyte Ca2+signals versus time and Ca2+area index after ChR2 stimulation (n=33 astrocytes from three mice). ***P<0.001; Wilcoxon test. Scale bar, 8%, 120 s. (d,e) Schematic drawing of targeted cell-attached recordings from GFP+excitatory neurons, and tdTomato-PV+neuronsin vivo, and the corresponding spike waveforms and fluorescence images. Astrocytes are depicted in red. Scale bars, 40 μm. (f,g) Cell-attached recordings showing the increase in spontaneous firing rate after astrocyte photostimulation.Bottom, corresponding histograms of number of spikes (bin width 10 s) versus time of the excitatory cell and PV+neuron (20 Hz, 2 min; blue bar) recorded ind,e, respectively. Scale bars, 1 mV, 60 s. (h,i) Histograms of firing rate changes after astrocyte stimulation for GFP+excitatory cells (n=45 from 25 mice, green) and PV+neurons (n=18 from 12 mice, red).Inset, normalized mean population spike waveform. Dark green, light green/red and white bars denote cells with a decrease, increase and no significant change in firing rate, respectively. (j) Relative changes of spontaneous firing rate before (control), after astrocyte stimulation and 10-min post stimulation (recovery). *P<0.05; two-tailed Student’st-test. Error bars indicate s.e.m. Figure 4: Astrocytes modulate spontaneous activity of PV + and excitatory visual cortex neurons in vivo . ( a ) Schematic illustration of the visual pathway in mice, and in vivo ChR2–mCherry expression in V1 for calcium imaging and electrophysiological recordings. ( b ) Representative fluorescence images of ChR2–mCherry-expressing astrocytes bulk-loaded with OGB (arrows). Scale bar, 40 μm. ( c ) Up , representative astrocyte Ca 2+ signals evoked by ChR2 stimulation (5 Hz, 20 s; blue bar). Scale bar, 40%, 60 s. Down , population astrocyte Ca 2+ signals versus time and Ca 2+ area index after ChR2 stimulation ( n =33 astrocytes from three mice). *** P <0.001; Wilcoxon test. Scale bar, 8%, 120 s. ( d , e ) Schematic drawing of targeted cell-attached recordings from GFP + excitatory neurons, and tdTomato-PV + neurons in vivo , and the corresponding spike waveforms and fluorescence images. Astrocytes are depicted in red. Scale bars, 40 μm. ( f , g ) Cell-attached recordings showing the increase in spontaneous firing rate after astrocyte photostimulation. Bottom , corresponding histograms of number of spikes (bin width 10 s) versus time of the excitatory cell and PV + neuron (20 Hz, 2 min; blue bar) recorded in d , e , respectively. Scale bars, 1 mV, 60 s. ( h , i ) Histograms of firing rate changes after astrocyte stimulation for GFP + excitatory cells ( n =45 from 25 mice, green) and PV + neurons ( n =18 from 12 mice, red). Inset , normalized mean population spike waveform. Dark green, light green/red and white bars denote cells with a decrease, increase and no significant change in firing rate, respectively. ( j ) Relative changes of spontaneous firing rate before (control), after astrocyte stimulation and 10-min post stimulation (recovery). * P <0.05; two-tailed Student’s t- test. Error bars indicate s.e.m. Full size image To study whether the astrocyte-mediated increase in inhibitory activity was a general property of all inhibitory neurons [27] , [28] , we also recorded SOM + neurons (in SOM-tdTomato mice; Fig. 5 ). In contrast to PV + neurons, SOM + neurons as a population showed no change in their overall spontaneous activity after astrocyte photostimulation ( Fig. 5b,d ). However, individual SOM + neurons displayed a wide range of effects from reduction to enhancement of their firing rate ( Fig. 5c ), indicating that astrocyte activation influences different subtypes of inhibitory neurons and their circuits in different ways in vivo , with consistent enhancement of activity only in a particular subset of inhibitory neurons—that is, PV + neurons. Cortical circuits enable neurons to integrate excitatory and inhibitory inputs, and the altered spontaneous activity of specific neurons in vivo likely reflects the balance of increased excitation and inhibition on them. 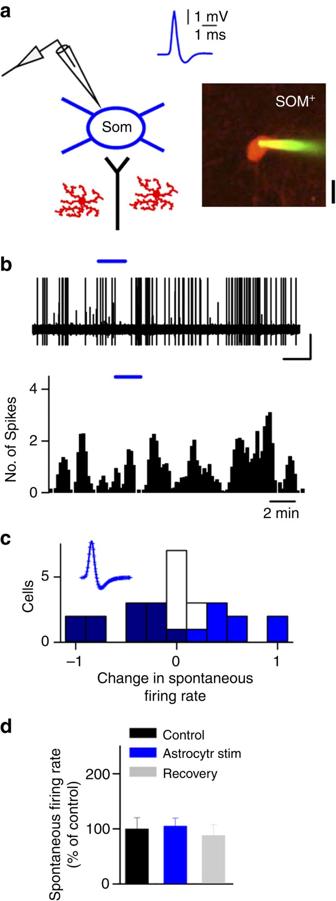Figure 5: Astrocytes induce changes in spontaneous activity of SOM+neuronsin vivo. (a) Schematic drawing of targeted cell-attached recordings in SOM+interneuronin vivo, and the corresponding spike waveform and fluorescence image. Astrocytes are labelled in red. Scale bar, 40 μm. (b) Spontaneous activity of cell-attached recordings inashowing no changes in the spontaneous firing rate after photostimulation of astrocytes (20 Hz for 2 min; blue bar). Bottom, corresponding histogram of number of spikes (bin width 10 s) versus time. Scale bar, 0.5 mV, 2 min. (c) Histogram of firing rate changes after astrocyte stimulation for SOM+neurons (n=27 from 14 mice). Dark blue, light blue and white bars denote cells with a decrease (n=11), increase (n=8) and no significant changes in firing rate (n=8), respectively. Inset, normalized mean population spike waveform. (d) Relative changes of spontaneous firing rate before (control), after astrocyte stimulation and 10-min post stimulation (recovery) (n=27). Error bars indicate s.e.m. Figure 5: Astrocytes induce changes in spontaneous activity of SOM + neurons in vivo . ( a ) Schematic drawing of targeted cell-attached recordings in SOM + interneuron in vivo , and the corresponding spike waveform and fluorescence image. Astrocytes are labelled in red. Scale bar, 40 μm. ( b ) Spontaneous activity of cell-attached recordings in a showing no changes in the spontaneous firing rate after photostimulation of astrocytes (20 Hz for 2 min; blue bar). Bottom, corresponding histogram of number of spikes (bin width 10 s) versus time. Scale bar, 0.5 mV, 2 min. ( c ) Histogram of firing rate changes after astrocyte stimulation for SOM + neurons ( n =27 from 14 mice). Dark blue, light blue and white bars denote cells with a decrease ( n =11), increase ( n =8) and no significant changes in firing rate ( n =8), respectively. Inset, normalized mean population spike waveform. ( d ) Relative changes of spontaneous firing rate before (control), after astrocyte stimulation and 10-min post stimulation (recovery) ( n =27). Error bars indicate s.e.m. Full size image Astrocytes drive changes in visual features of V1 neurons If astrocyte activation alters excitatory and inhibitory activities in cortical circuits, then the response selectivity of cortical neurons that relies on integration of this activity [29] , [30] , [31] could also be affected. We thus investigated whether astrocyte signalling could drive changes in the key visual response features of V1 neurons. Specifically, we examined stimulus-driven (ON minus OFF) responses of neurons to oriented drifting gratings, and derived parameters that describe the tuning properties of these neurons ( Supplementary Fig. 5a ). Light stimulation of V1 in mice without GFAP-ChR2 infection had no effect on any of the properties of V1 neurons ( Supplementary Fig. 5 ). However, in ChR2-infected mice, light stimulation caused a selective enhancement in the baseline firing rate of PV + neurons, a parameter independent of spontaneous activity that measures the overall level of visually driven responses (0.71±0.30 Hz pre- versus 1.80±0.54 Hz post-astrocyte stimulation; P =0.008 Wilcoxon test; n =18; Fig. 6b,c ). An increase in the baseline predicts a reduction in specific tuning parameters such as the Orientation Selectivity Index (OSI; Supplementary Fig. 5a , see Methods Equation (2)) but little change in complementary parameters such as the tuning width. PV + cells with a significant change in the baseline showed a robustly reduced OSI after astrocyte photostimulation (0.46±0.05 pre- versus 0.30±0.05 post-astrocyte stimulation; P <0.001, Wilcoxon test; n =14; Fig. 6d ), with no major changes in other parameters ( Fig. 6d and Supplementary Fig. 6a ). On the other hand, most excitatory cells displayed complex responses to astrocyte stimulation, showing either an increase or decrease in their baseline firing rate ( Fig. 7b,c ; n =45), consistent with changes in net excitatory and inhibitory drive on them. As predicted, changes in baseline were inversely related to changes in orientation and direction selectivity ( Supplementary Fig. 6b ). Excitatory cells that showed an increase in their baseline activity (0.07±0.04 Hz pre- versus 0.17±0.07 Hz post-astrocyte stimulation; P =0.015, Wilcoxon test; 16 out of 36 significantly affected cells), displayed a reduction in their OSI (0.59±0.06 pre- versus 0.39±0.06 post-astrocyte stimulation; P <0.001, Wilcoxon test) and Direction Selectivity Index (DSI, 0.55±0.07 pre- versus 0.35±0.05 post-astrocyte stimulation; P =0.02, Wilcoxon test; Fig. 7d,e ; see Methods Equation (3)). In contrast, excitatory cells that showed a reduction in baseline activity (0.16±0.06 Hz pre- versus 0.04±0.02 Hz post-astrocyte stimulation; P =0.007, Wilcoxon test; 20 out of 36 significantly affected cells) expressed an increase in their OSI (0.50±0.05 pre- versus 0.67±0.05 post-astrocyte stimulation; P =0.008, Wilcoxon test) and DSI (0.53±0.05 pre- versus 0.66±0.07 post-astrocyte stimulation; P =0.04, Wilcoxon test; Fig. 7f,g ). In both cases, astrocyte stimulation did not evoke significant changes in tuning width, preferred orientation (PO) or peak firing rate ( Figs 6e and 7e,g and Supplementary Fig. 6a,b ). Although astrocytes controlled both spontaneous firing rate ( Fig. 4 ) and visually evoked responses of PV + and excitatory neurons ( Figs 6 and 7 ), no causal link was found between these two parameters ( Supplementary Fig. 6c,d ), indicating that changes in stimulus selectivity resulted from the influence of astrocytes on visually active synapses rather than on nonspecific background activity. Thus, astrocyte activation increases baseline visual responses of PV + neurons and reduces their orientation selectivity but not direction selectivity, likely due to the very low control direction selectivity of these cells ( Fig. 6d,e ) [32] , [33] . In turn, astrocyte activation alters the baseline and the orientation and direction selectivity of excitatory neurons, in an inverse and systematic relationship to their change in baseline. 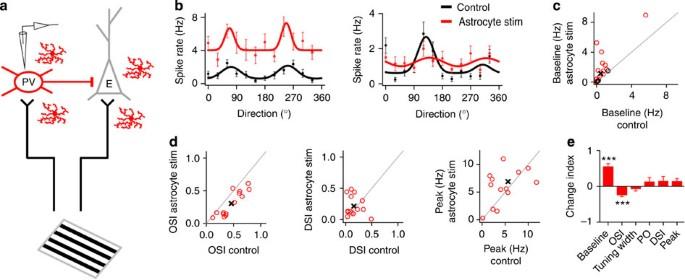Figure 6: Astrocytes induce changes in visual response properties of PV+neuronsin vivo. (a) Schematic drawings of cell-attached recordings from PV+neuron, visual stimulation, putative intracortical connectivity and ChR2-transfected astrocytes. (b) Representative tuning curves of two PV+neurons before (Control, black) and after astrocyte stimulation (red). Tuning curves are best-fit Gaussians to the mean firing rates (dots denote measured firing rates and lines denote fitted curves; error bars denote s.e.m. of 10 responses). (c) Population summary of astrocyte-induced changes in baseline firing rate (circles denote individual cells,n=18. Black circles, cells with no significant changes that were discarded from subsequent analyses,n=4. Cross denotes population average). (d) Population summary of astrocyte-induced changes in OSI, DSI and peak firing rate (n=14). (e) Index (normalized change) in tuning properties after versus before astrocyte stimulation. ***P<0.001; Wilcoxon test. Error bars indicate s.e.m. Figure 6: Astrocytes induce changes in visual response properties of PV + neurons in vivo. ( a ) Schematic drawings of cell-attached recordings from PV + neuron, visual stimulation, putative intracortical connectivity and ChR2-transfected astrocytes. ( b ) Representative tuning curves of two PV + neurons before (Control, black) and after astrocyte stimulation (red). Tuning curves are best-fit Gaussians to the mean firing rates (dots denote measured firing rates and lines denote fitted curves; error bars denote s.e.m. of 10 responses). ( c ) Population summary of astrocyte-induced changes in baseline firing rate (circles denote individual cells, n =18. Black circles, cells with no significant changes that were discarded from subsequent analyses, n =4. Cross denotes population average). ( d ) Population summary of astrocyte-induced changes in OSI, DSI and peak firing rate ( n =14). ( e ) Index (normalized change) in tuning properties after versus before astrocyte stimulation. *** P <0.001; Wilcoxon test. Error bars indicate s.e.m. 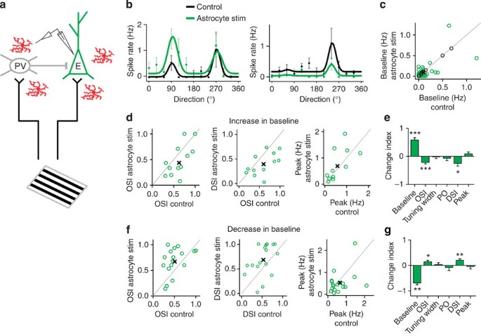Figure 7: Astrocytes drive changes in visual response properties of excitatory neuronsin vivo. (a) Schematic drawings of cell-attached recordings from excitatory neuron, visual stimulation, putative intracortical connectivity and ChR2-transfected astrocytes. (b) Representative tuning curves of two excitatory neurons before (Control, black) and after astrocyte stimulation (green). (c) Population summary of astrocyte-induced changes in baseline firing rate (circles denote individual cells,n=45. Black circles, cells with no significant changes that were discarded from subsequent analyses,n=9). (d,f) Population summary of astrocyte-induced changes in OSI, DSI and peak firing rate of cells with an increase (d;n=16) or decrease (f;n=20) in baseline. (e,g) Index (normalized change) in tuning properties after versus before astrocyte stimulation for cells with an increase (e;n=16) or decrease (g;n=20) in baseline. *P<0.05, **P<0.01, ***P<0.001; Wilcoxon test. Error bars indicate s.e.m. Full size image Figure 7: Astrocytes drive changes in visual response properties of excitatory neurons in vivo . ( a ) Schematic drawings of cell-attached recordings from excitatory neuron, visual stimulation, putative intracortical connectivity and ChR2-transfected astrocytes. ( b ) Representative tuning curves of two excitatory neurons before (Control, black) and after astrocyte stimulation (green). ( c ) Population summary of astrocyte-induced changes in baseline firing rate (circles denote individual cells, n =45. Black circles, cells with no significant changes that were discarded from subsequent analyses, n =9). ( d , f ) Population summary of astrocyte-induced changes in OSI, DSI and peak firing rate of cells with an increase ( d ; n =16) or decrease ( f ; n =20) in baseline. ( e , g ) Index (normalized change) in tuning properties after versus before astrocyte stimulation for cells with an increase ( e ; n =16) or decrease ( g ; n =20) in baseline. * P <0.05, ** P <0.01, *** P <0.001; Wilcoxon test. Error bars indicate s.e.m. Full size image Visual responses were also recorded in SOM + neurons. Astrocyte stimulation evoked changes in the baseline firing rate of SOM + cells ( Fig. 8 ); however, rather than uniformly increasing their baseline visual responses similar to PV + neurons, SOM + neurons showed either a decrease (12 out of 27 neurons) or an increase of the baseline (10 out of 27 neurons; Fig. 8c ). Changes in baseline were accompanied by significant complementary changes in OSI ( Fig. 8d–g ; Supplementary Fig. 7 ). Taken together, these results indicate that astrocytes have an impact on the tuning properties of V1 cortical neurons, affecting consistently the baseline of PV + interneurons but with variable effects on excitatory cells and SOM + interneurons. 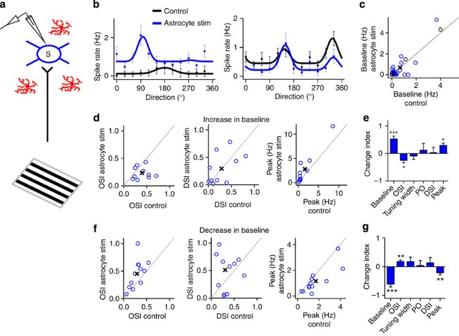Figure 8: Astrocytes induce changes in visual response properties of SOM+neuronsin vivo. (a) Schematic drawing of targeted cell-attached recordings in SOM+interneuron, visual stimulation and ChR2-transfected astrocytes. (b) Representative tuning curves of two SOM+neurons before (Control, black) and after astrocyte stimulation (blue). Dots denote measured firing rates and lines denote fitted curves (error bars denote s.e.m. of 10 responses). (c) Population summary of astrocyte-induced changes in baseline firing rate (circle, individual cell;n=27 from 14 mice. Black circles, cells with no significant changes,n=5. Cross, population average). (d,f) Population summary of astrocyte-induced changes in OSI, DSI and peak firing rate from cells that displayed an increase (d;n=10) or decrease (f;n=12) in baseline firing rate. (e,g) Index (normalized change) in tuning properties after versus before astrocyte stimulation for cells with an increase (e;n=10) or decrease (g;n=12) in baseline. *P<0.05; **P<0.01; ***P<0.001; Wilcoxon test. Error bars indicate s.e.m. Figure 8: Astrocytes induce changes in visual response properties of SOM + neurons in vivo . ( a ) Schematic drawing of targeted cell-attached recordings in SOM + interneuron, visual stimulation and ChR2-transfected astrocytes. ( b ) Representative tuning curves of two SOM + neurons before (Control, black) and after astrocyte stimulation (blue). Dots denote measured firing rates and lines denote fitted curves (error bars denote s.e.m. of 10 responses). ( c ) Population summary of astrocyte-induced changes in baseline firing rate (circle, individual cell; n =27 from 14 mice. Black circles, cells with no significant changes, n =5. Cross, population average). ( d , f ) Population summary of astrocyte-induced changes in OSI, DSI and peak firing rate from cells that displayed an increase ( d ; n =10) or decrease ( f ; n =12) in baseline firing rate. ( e , g ) Index (normalized change) in tuning properties after versus before astrocyte stimulation for cells with an increase ( e ; n =10) or decrease ( g ; n =12) in baseline. * P <0.05; ** P <0.01; *** P <0.001; Wilcoxon test. Error bars indicate s.e.m. Full size image Consistent with changes in excitatory/inhibitory synaptic transmission mediated by mGluR1a activation in slices ( Figs 2 and 3 ), systemic administration of AIDA (5 mg kg −1 intraperitoneal, a selective antagonist of mGluR1a) blocked the astrocyte-induced changes in baseline and OSI in excitatory cells and PV + neurons ( Fig. 9 ), indicating that astrocyte activity in vivo regulates visual tuning properties of cortical neurons through mGluR1a activation. 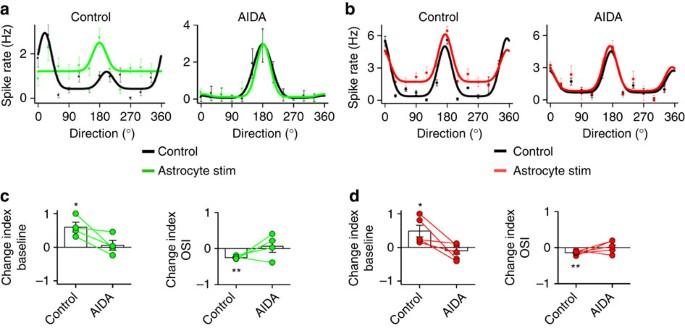Figure 9: Astrocyte-induced changes of visual features in cortical neurons are mediated by mGluR1a activation. (a) Tuning curves of an excitatory neuron before (Control, black) and after astrocyte stimulation (green), in control and 30 min after intraperitoneal injection of AIDA (5 mg kg−1). Dots denote measured firing rates and lines denote fitted curves (n=10 responses). (b). Tuning curves of a PV+neuron before (Control, black) and after astrocyte stimulation (red), in control and after AIDA injection. (c) Summary of astrocyte-induced changes in baseline firing rate and OSI in excitatory cells (circle, individual cell. Bars, average data;n=4 from four mice) (d) Summary of astrocyte-induced changes in baseline firing rate and OSI in PV+neurons (circle, individual cell. Bars, average data;n=5 from five mice). The changes observed after astrocyte stimulation were abolished in the presence of mGluR1a antagonist, AIDA. *P<0.05; **P<0.01; Wilcoxon test. Error bars indicate s.e.m. Figure 9: Astrocyte-induced changes of visual features in cortical neurons are mediated by mGluR1a activation. ( a ) Tuning curves of an excitatory neuron before (Control, black) and after astrocyte stimulation (green), in control and 30 min after intraperitoneal injection of AIDA (5 mg kg −1 ). Dots denote measured firing rates and lines denote fitted curves ( n =10 responses). ( b ). Tuning curves of a PV + neuron before (Control, black) and after astrocyte stimulation (red), in control and after AIDA injection. ( c ) Summary of astrocyte-induced changes in baseline firing rate and OSI in excitatory cells (circle, individual cell. Bars, average data; n =4 from four mice) ( d ) Summary of astrocyte-induced changes in baseline firing rate and OSI in PV + neurons (circle, individual cell. Bars, average data; n =5 from five mice). The changes observed after astrocyte stimulation were abolished in the presence of mGluR1a antagonist, AIDA. * P <0.05; ** P <0.01; Wilcoxon test. Error bars indicate s.e.m. Full size image We have shown that stimulation of astrocytes increases excitatory synaptic transmission to layer 2/3 excitatory and inhibitory neurons in V1 cortical slices through the activation of presynaptic mGluR1a. Astrocytes in vivo drive changes in the basal tone of V1 cortical activity, increasing the spontaneous firing rate of PV + neurons and either increasing or decreasing the spontaneous rate of excitatory and SOM + neurons. Moreover, astrocyte stimulation strongly influences the visual responses of V1 neurons, selectively increasing the baseline level of visual drive to PV + neurons and reducing their orientation selectivity, while altering net excitatory/inhibitory drive to excitatory and SOM + neurons and influencing both their baseline levels and orientation and direction selectivity. These effects are consistent with the circuits formed by these neurons. PV + neurons receive strong feedforward drive and provide direct perisomatic inhibition on target excitatory neurons [30] , [31] , [32] , which also receive monosynaptic inhibition from SOM + neurons [34] . SOM + neurons integrate widespread inputs from cortical excitatory neurons [35] and also receive inhibitory connections from other interneurons, such as vasoactive intestinal peptide (VIP + )-expressing neurons [34] . Therefore, by enhancing excitatory drive to excitatory and inhibitory neurons, astrocyte activation can drive changes in diverse information-processing circuits of visual cortex. By inducing with ChR2 levels of astrocyte activity that can be evoked by natural (visual) stimuli, we have shown a modulatory role of astrocytes in sensory information processing. Ideally, to definitively unmask the contribution of astrocytes to cortical operations in normal vision, visually driven Ca 2+ responses of astrocytes should be transiently blocked; unfortunately, currently available tools are not specific or fast enough to prevent physiological astrocyte Ca 2+ signalling in vivo (for example, astrocyte-specific deletion of IP3R2-mediated Ca 2+ responses in IP3R2 knockout mice [8] , [12] or local application of the Ca 2+ chelator 1,2-bis( o -aminophenoxy)ethane- N,N,N′,N′ -tetraacetic acid (BAPTA) [34] fail to transiently and selectively block astrocyte Ca 2+ signals in vivo , respectively, while electrical activity of single cortical neurons are recorded). Here using optogenetics we focused our study on boosting astrocyte signalling to reveal their contribution to cortical network operations. Optogenetic manipulation of astrocytes with ChR2 is still a novel method to activate astrocytes [14] , [22] ; we have shown the contribution of the intracellular stores to the ChR2 Ca 2+ -induced responses in astrocytes ( cf , ref. 14 ), and the physiological consequences of astrocyte activation in regulating specific response features of sensory cortex neurons in vivo . Given the functional significance of the temporal and spatial properties of astrocyte Ca 2+ signalling on neuronal physiology, whether local or individual ChR2-astrocyte stimulation could evoke subtle changes in synaptic transmission, as has been previously described for evoked EPSCs at single synapses [3] , [6] , [17] , [26] , is still unresolved. Therefore, many questions remain open and further studies are required to fully understand the molecular mechanisms underlying the ChR2-induced Ca 2+ elevations in astrocytes and their relevance for other brain functions. Despite these caveats, our findings support an integral role for astrocytes in basal transmission and configuration of neuronal responses. They complement previous in vivo results showing that transient blockade of astrocyte glutamate transporters [9] or astrocyte-specific deletion of IP3R2-mediated Ca 2+ responses [8] prolongs the orientation-tuning response [9] and abolishes adaptation-induced changes in orientation-tuning curves [8] , respectively. As alterations in excitatory and inhibitory drive influence not only the response level and feature selectivity of neurons but also the coding and transmission of information [36] , [37] , and the representation and integration of information in neuronal populations [38] , [39] , changes in excitatory and inhibitory transmissions by astrocyte activity suggest that astrocytes would be involved in multiple aspects of information coding by cortical circuits. Indeed, astrocytes, through the specific activation of PV + interneurons, could act as an important cellular influence on a range of cortical functions, such as circuit and columnar development [40] and feedforward control of response gain and selectivity [30] , [31] , [41] , [42] . Mice All experiments were performed under protocols approved by the Animal Care and Use Committee at MIT and conformed to the NIH guidelines. Wild-type and transgenic line mice used for in vivo and slice experiments included the following: C57BL/6 wild-type mice, thy1-GFP-S (Jackson Labs), heterozygous PV-Cre knockin driver mice [32] and SOM-Cre knockin driver mice [43] backcrossed to a Cre-responsive reporter line (Ai9-lsl-tdTomato transgenic mice [44] ; Jackson Labs). ChR2 virus injection ChR2 fused to mCherry (ChR2–mCherry; provided by Dr Boyden) was cloned into adeno-associated virus (AAV) particles (serotype 5; UNC) using the GFAP promoter GFAP104 (AAV2.5-GFAP-ChR2–mCherry). To prepare animals for in vivo experiments, 5- to 6-week-old male and female wild-type and transgenic mice were initially anaesthetized with 4% isoflurane in oxygen, and maintained on 2% isoflurane. The target coordinates were displaced from Bregma by 3.5 mm posterior and 2.2 mm lateral. The skull was thinned along a 1-mm line at the rostral edge of V1, and the remaining skull and dura were punctured using a glass micropipette filled with the virus. Two injections were made at each site, one at 400 μm below the cortical surface, and one at a depth of 250 μm. A volume of 0.3 μl of virus was injected at 50 min −1 at each depth. After each injection, the pipette was held in place for 5 min before retraction to prevent leakage. Following injection, the micropipette was removed, the folded skull replaced and the skin sutured with 6–0 vicryl suture. The animal was allowed to recover from anaesthesia with the help of heating pads and was returned to the cage once it showed regular breathing and locomotion. For slice experiments that were performed after 2 weeks of viral injection, neonatal wild-type, PV-tdTomato and SOM-tdTomato mice (P5) were anaesthetized by immersion in ice for 1–2 min. Animals were covered with gauzes immersed in cold water to maintain anaesthesia levels and placed in a custom-made stereotactic apparatus. The overall duration of this procedure was kept under 20 min so as to maximize the survival rate of the pups. After 2 weeks of survival, we confirmed with immunostaining that mCherry expression was specific to astrocytes ( Fig. 1a ). In core regions of infection, GFAP staining and mCherry expression colocalized in astrocytes, while no colocalization was observed in NeuN-labelled neurons ( Supplementary Fig. 3 ). Electrophysiology in slices Two weeks after viral injection, ~P20 male and female C57BL/6 wild-type, PV-tdTomato and SOM-tdTomato mice were anaesthetized and decapitated. The brain was rapidly removed and placed in ice-cold artificial cerebrospinal fluid (ACSF). Cortical slices (300 μm thick) were incubated for >1 h at room temperature (21–24 °C) in ACSF that contained (in mM): NaCl 124, KCl 2.69, KH 2 PO 4 1.25, MgSO 4 2, NaHCO 3 26, CaCl 2 2 and glucose 10, and was gassed with 95% O 2 /5% CO 2 (pH=7.3). Slices were then transferred to an immersion-recording chamber and superfused with gassed ACSF. Cells were visualized with an Olympus BX50WI microscope (Olympus Optical, Tokyo, Japan) coupled with a × 40 water immersion lens, infrared-DIC optics and MetaFluor software (Molecular Devices, LLC)-driven infrared Coolsnap cf2 CCD camera (Photometrics). Whole-cell patch-clamp recordings from layer 2/3 neurons were obtained with an Axopatch 200B amplifier (Molecular Devices, LLC). Patch electrodes (3–5 MΩ) were filled with internal solution that contained (in mM) for EPSC recordings: KGluconate 135, KCl 10, HEPES 10, MgCl 2 1, ATP-Na 2 2, titrated with KOH to pH 7.3. For IPSC recordings patch electrodes were filled with the following: CsCl 130, NaCl 1, MgCl 2 1, CaCl 2 1, EGTA 5, HEPES 10, ATP-Na 2 2, GTP-Na 0.2 and QX-314 5, titrated with CsOH to pH=7.3 (ref. 45 ). For the IPSC recordings, the chloride equilibrium potential was 0.83 mV. Recordings were rejected when the access resistance increased >20% during the experiment. Signals were fed to a Pentium-based PC through a DigiData 1,440 interface board (Molecular Devices, LLC). The pCLAMP 10.2 software (Molecular Devices, LLC) was used for data display, acquisition and storage. Experiments were performed at room temperature (21–24 °C). Cells were voltage-clamped at −60 mV. ACSF included bicuculline (10 μM) for EPSC recordings and TTX (1 μM) for mEPSCs. NBQX (20 μM) and APV (50 μM) were used for spontaneous IPSCs, plus TTX (1 μM) for mIPSC recordings. In a subset of experiments, IPSCs were blocked by application of bicuculline (10 μM). Experiments designed to optimize NMDA receptor activation and recording slow inward currents were performed in a modified Mg 2+ -free ACSF (Mg 2+ was equimolarly substituted by Ca 2+ ) plus TTX (1 μM). Drugs were bath-applied (for indicated experiments drugs were applied for at least 15 min before recordings). Electrophysiological responses were measured 5 min before astrocyte stimulation (Control), during and up to 5 min of astrocyte stimulation (Astrocyte stim), and after 10–15 min of stimulation (Recovery). Control experiments were performed in V1 slices from the non-infected hemisphere to examine the specificity of the observed responses to astrocyte ChR2-induced stimulation. For slice recordings, one neuron was recorded per slice and two to three slices were recorded per mouse. Analysis of slow currents Both the spontaneous and ChR2-induced slow inward currents were discriminated from standard mEPSCs based on their time courses—that is, rise and decay time ( Fig. 2b ). The time course analysis of mEPSCs and slow inward currents showed that rise and decay times were significantly faster for mEPSC than for slow inward currents. Rise time: 3.66±0.33 ms for mEPSC; 18.64±2.31 ms for SIC ( P <0.001, t -test). Decay time: 18.48±1.42 ms for mEPSC; 46.04±3.42 ms for SIC ( n =28; P <0.001, t -test). No differences were found between spontaneous and ChR2-induced slow currents: rise time 17.77±1.60 ms for spontaneous, 19.19±3.71 ms for ChR2-evoked ( P =0.97, t -test); decay time 41.55±5.08 ms for spontaneous, 48.85±4.38 ms for ChR2-evoked ( n =10 neurons; P =0.95, t -test). Values denote mean±s.e.m. To avoid possible controversies regarding the definition of slow inward currents, we used criteria described previously in the hippocampus [18] , [19] , [20] and visual cortex [8] . Calcium imaging in slices Calcium signals from layer 2/3 astrocytes were monitored by fluorescence microscopy using the Ca 2+ indicator Fura-2 (Molecular Probes, Eugene, OR, USA). Slices were pre-incubated in ACSF containing 1 mM Fura-2 AM, 0.4% pluronic F-127 in DMSO and 95% O 2 /5% CO 2 for 30 min at room temperature, and then they were rinsed in fresh ACSF and transferred to the slice chamber. Astrocytes were illuminated for 100–300 ms with a xenon lamp at 490 nm using Lambda DG4 illumination system (Sutter Instruments, Novato, CA, USA) and images were acquired every 1–2 s. The illumination and CCD camera were controlled and synchronized using the MetaFluor software (Molecular Devices, LLC) that was also used for ratiomeric epifluorescence measurements. Ca 2+ levels were recorded from the cell body of mCherry-positive astrocytes and Ca 2+ variations were estimated as changes in the 380/340 ratio over the baseline. Astrocytes were considered to respond to the stimulation when 380/340 ratio increased two times the s.d. of the baseline for at least two consecutive images and with a delay ⩽ 15 s after stimulation. Evoked responses were analysed by measuring the Calcium Area in 20 s bins before and after the stimulus: Calcium Area= F(t)dt; t 0, t i=zero time and the end of the recording, respectively; F=Ca 2+ fluorescence signal; t =time; d t =image acquisition rate in seconds. The Calcium Area Index was calculated as: [(Area_postStim)−(Area_preStim)]/[(Area_postStim)+(Area_preStim)] (Equation (1)). Cells were not recorded for longer periods than 5 min after ChR stimulation. For control experiments, astrocyte Ca 2+ signals from naive V1 contralateral to the infected hemisphere were recorded before and after blue-light stimulation. In a subset of experiments, ATP (20 mM) was applied by pressure injection to monitor the calcium responses of naive astrocytes ( Supplementary Fig. 4a ). Dissociated astrocyte cultures Primary astrocyte cultures were prepared from cerebral cortices of Swiss Webster mice (P0-P1; Charles River) through a protocol modified from that used previously [46] . Briefly, approximately ¼ of cortex was isolated and treated with trypsin (1 mg ml −1 ) for 13 min at room temperature. Digestion was stopped by Hanks solution supplemented with 10% fetal bovine serum and trypsin inhibitor. Tissue was dissociated with silicone-coated Pasteur pipettes and centrifuged at 1,000 r.p.m. at 4 C° for 10 min. Dissociated cells were plated with plating medium (500 ml MEM, with 2.5 g D -glucose, 50 mg transferrin, 5 ml of L -glutamine and 50 ml fetal bovine serum) on glass coverslips precoated with Matrigel (BD Biosciences). Then, for every 12 wells, 12 μl AAV-GFAP104-ChR2–mCherry virus was added to 1.2-ml plating medium, mixed well and 100 μl virus mixture was added to each well. After 7–10 days of virus expression, cells were used for experiments. Cells were visualized and recorded with a Zeiss LSM 510 confocal microscope and MetaMorph software (Molecular Devices, LLC); an optical switch with xenon lamp (Sutter Instruments, as above) was used to deliver light pulses for ChR2 activation and Fura-2 calcium recordings. In vivo preparation For the in vivo experiments, two-photon calcium imaging and cell-attached recordings were performed on 7- to 8-week-old C57BL/6 mice and transgenic mice. After 2 weeks of post-injection survival, to ensure a high level of transgene expression, mice were anaesthetized with a cocktail containing fentanyl (0.05 mg kg −1 ), midazolam (5 mg kg −1 ) and medetomidine (0.5 mg kg −1 ) and maintained with 0.2–0.5% isoflurane as necessary. Atropine sulphate (5 mg kg −1 ) was intraperitoneally injected. Ophthalmic ointment was used to protect the animal’s eyes during the surgery and replaced with silicon oil during recordings. Body temperature was maintained at 37.5 °C with a heating blanket (Harvard Apparatus). A metal headplate was attached to the skull with cyanoacrylate glue and dental acrylic. A 2 × 2 mm craniotomy was made over the primary visual cortex (V1), which was later covered with a thin layer of 2% agarose in ACSF (140 mM NaCl, 5 mM KCl, 2 mM CaCl 2 , 1 mM MgCl 2 , 0.01 mM EDTA, 10 mM HEPES, 10 mM glucose, pH 7.4). The headplate was then screwed into a moveable stage and transferred to the microscope (described below), 0.5% isoflurane in oxygen was supplied and fentanyl/medetomidine injected as needed every few hours. In vivo two-photon calcium imaging A glass pipette filled with 1.0 mM Oregon Green-488 Bapta-1-AM (OGB1-AM; Molecular Probes) was visually guided into layer 2/3 using a micromanipulator (Sutter Instruments, MP-285) and a small volume was pressure-injected using a Picospritzer. In vivo imaging of OGB1-AM signals in mCherry-expressing astrocytes was performed with a two-photon laser scanning microscope at excitation wavelength 810 nm (Prairie Technologies, Spectra Physics Mai-Tai eHP laser passed through a Deep-See module; Spectra Physics/Newport). Fluorescence was detected using photomultiplier tubes (R6357; Hamamatsu, Japan). A × 25, 0.95 NA lens (Olympus Optical) was used. Imaged cells were located at a depth of 100–200 μm below the pial surface. Custom-written software in Matlab was used for computation of the time-lapse ΔF/F for each distinct region of interest (ROI). Astrocytes were discriminated from neurons by mCherry labelling, and their ROIs were manually selected on the OGB1-AM fluorescence image. The raw fluorescence intensity was smoothed with a Gaussian kernel, and the change in fluorescence normalized by the baseline fluorescence (ΔF/F) was computed for each ROI. The baseline fluorescence was defined as the average fluorescence across pre-stimulus frames, while the change in fluorescence was computed as the baseline fluorescence subtracted from the maximum fluorescence intensity during the stimulus (ChR2 or visual stimulation). Evoked responses were analysed by measuring the calcium area in 20-s bins before and after ChR2 or visual stimulation, and the Calcium Area Index was calculated (see Equation (1)). Cells were not recorded for longer periods than 5 min after ChR stimulation. In vivo cell-attached recording For fluorescent visualization, glass pipettes (1.5 mm tip size, 3–7 MΩ) were filled with Alexa Fluor 488 (100 um, Molecular Probes) or Alexa Fluor 594 (100 um, Molecular Probes) and held at positive pressure. The pipette was targeted to the injection site using a × 10 lens, and then targeted to individual cells using a × 25 lens via concurrent two-photon imaging at 770 or 920 nm to 100–200 μm below the pial surface (layer 2/3) using a micromanipulator [32] . Cells were either targeted by moving the pipette into their vicinity and then commencing diagonal advance, or cells were patched blindly by advancing diagonally through the cortex. The resistance of the pipette was monitored during the penetration by delivering −0.5 nA current pulses for 6.3 ms at 0.55 Hz with a Multiclamp amplifier and Clampex 10.2 software (Molecular Devices, LLC). When a seal with a cell during the advancement of pipette was obtained (assessed by increase in pipette tip resistance) and well-isolated spikes were detected during visual stimuli presentation, sustained negative pressure was applied (0.2–0.6 psi) to secure the seal [47] . Recordings were performed at a sampling rate of 20 kHz and filtered between 300 Hz and 5 kHz. The pClamp data were analysed with Clampfit 10.2 software (Molecular Devices, LLC) and Matlab with custom-written scripts to calculate firing rates in epochs with and without visual stimulus presentation. Blind cell-attached recordings were performed in wild-type mice. Two-photon-guided targeted cell-attached recordings were performed in thy1-GFP-S (for GFP + excitatory cells), PV-tdTomato (for PV + interneurons) and SOM-tdTomato transgenic mice (for SOM + interneurons) to confirm the cellular type and their specific responses to astrocyte stimulation. Visual stimulation and data analysis Visually driven responses and tuning properties were evaluated in layer 2/3 neurons. Visual stimuli, generated with the Psychophysics toolbox [48] in Matlab, were displayed on a 19-inch LCD monitor situated 15 cm from the eyes. The onset of the visual stimulus was synchronized to the initiation of acquisition of two-photon calcium images and cell-attached recordings. In the calcium imaging experiments, the visual stimuli consisted of random orientation square wave drifting grating stimuli at 100% contrast in 12 randomly permuted directions, each 30 degrees apart and lasting for 666 ms. This stimulus was presented for 8 s alternating with a blank grey screen for 30 s across multiple cycles. Episodic orientated grating stimuli were applied while cell-attached recordings from V1 neurons were performed. Gratings were then presented by stepping the orientation from 0 to 360 degrees in steps of 30 degrees. The duration of each grating presentation was 2 s ‘ON’ followed by 2 s ‘OFF’ (blank grey screen), with 12 s as resting period before the first grating, for a total duration of 60 s for one set of stimuli per ‘trial’. Each of these trials was then repeated with and without optogenetic stimulation at least 10 times. Gaussian fits (see Supplementary Fig. 5 ) were computed for the tuning curves using a sum of two Gaussians with peaks 180° apart and five parameters: PO, tuning width σ (computed as the half-width at half-maximum of the Gaussian function), baseline response (average level of activity above zero of the flat portion of the Gaussian), maximum response at the PO and direction (R(a)) and response at the non-preferred direction (R(b)) [49] . Optimal parameters were determined with least-squares fits. The OSI was computed by taking the vector average for the PO according to the formula OSI=sqrt[sum(response × cos(2 × theta)) 2 +sum(response × sin(2 × theta) 2 ))]/sum(responses) (Equation (2)). The DSI was calculated as: [R(a)−R(b)]/[R(a)+R(b)] (Equation (3)) (ref. 30 ). Baseline firing rate was independent of spontaneous activity and was calculated as ON minus OFF responses. The Pearson correlation coefficient ( r ) was used to quantify the relationship between the changes in tuning parameters. Cells were classified into two groups based on the effect of astrocytes on their baseline firing rate—that is, increase in baseline and decrease in baseline. Cells with no significant changes in baseline after astrocyte stimulation were discarded from the analysis for the rest of tuning parameters. Optogenetic stimulation Two weeks after viral injection, cells expressing mCherry, denoting functional ChR2 expression, were readily visualized. To drive these cells, we employed a diode-pumped solid-state blue laser with analogue intensity control (473 nm, 200 mW, MBL-III-473, OptoEngine, LLC) coupled via SMA terminal to a 200-μm fibre (ThorLabs) that was placed over the slices or over the cranial window in vivo for full-field stimulation. Blue-light pulses (2–5 mW, 20 ms) were delivered at 10–20 Hz. Light stimulus durations were adjusted and selected to evoke reliable astrocyte calcium signals and neuronal responses ( Supplementary Fig. 3 ). For in vivo astrocyte calcium imaging, blue-light stimulation was delivered through the light path of the two-photon microscope at 2–5 Hz for 20–30 s. For Ca 2+ recordings in astrocyte cultures, light pulses were delivered through the microscope light path at 20 Hz for variable durations ( Supplementary Fig. 2 ). Immunohistochemistry C57/BL6 mice transfected with AAV2.5-GFAP-ChR2–mCherry were overdosed with pentobarbital and perfused transcardially with saline followed by 4% paraformaldehyde ( n =3 mice). The brain was extracted and kept in paraformaldehyde overnight. The brain was sectioned in 50 μm slices that were then blocked in 10% normal goat serum with 1% triton in phosphate-buffered saline (1 h, room temperature) and stained for rabbit anti-GFAP (1:200, Sigma, G9269) and mouse anti-NeuN (1:250, Millipore, MAB377) overnight (<4 °C). This was followed by a 3-h incubation in Alexa Fluor 488 goat anti-rabbit (1:200, Invitrogen, A11034) and Alexa Fluor 405 goat anti-mouse (1:200, Invitrogen, A31553) before being mounted on a glass slide with the Vectashield Hardset mounting media (Vector Labs). The slides were imaged using a confocal microscope (Zeiss LSM 5 Pascal Exciter). Drugs and chemicals D -(-)-2-Amino-5-phosphonopentanoic acid (D-AP5), 2,3-Dioxo-6-nitro-1,2,3,4-tetrahydrobenzoquinoxaline-7-sulfonamide disodium salt (NBQX), bicuculline, Tetrodotoxin (TTX), N -(2,6-dimethylphenylcarbamoylmethyl)triethylammonium chloride (QX-314), (S)-α-Methyl-4-carboxyphenylglycine (MCPG), (S)-(+)-α-Amino-4-carboxy-2-methylbenzeneacetic acid (LY367385), (RS)-1-Aminoindan-1,5-dicarboxylic acid (AIDA) and Pyridoxalphosphate-6-azophenyl-2′,4′-disulphonic acid tetrasodium salt (PPADS) were purchased from Tocris Cookson (Bristol, UK). Fura-2 AM, Oregon Green-488 BAPTA-1-AM, Sulforhodamine101 (SR101), Alexa Fluor 488 and Alexa Fluor 594 were purchased from Molecular Probes. All other drugs were purchased from Sigma. AIDA (5 mg kg −1 ) was administered intraperitoneally and cell-attached recordings recommenced after a period of at least 30 min. Statistical analyses Data are presented as mean values±s.e.m. Statistical analyses of experiments to assess significance were conducted with two-tailed Student’s t -test ( α =0.05) or Wilcoxon-Signed Rank Test as appropriate. Statistical differences were established with * P <0.05, ** P <0.01 and *** P <0.001. How to cite this article: Perea, G. et al . Optogenetic astrocyte activation modulates response selectivity of visual cortex neurons in vivo . Nat. Commun. 5:3262 doi: 10.1038/ncomms4262 (2014).